Novel survey method finds dramatic decline of wild cotton-top tamarin population Although much of the world's focus has been on the disappearance of ape populations in Africa and Asia ( http://www.unep.org/grasp/ ), the plight of New World primates is of urgent global concern [1] . Cotton-top tamarins ( Saguinus oedipus ) are small arboreal monkeys (0.5 kg) of the family Callitrichidae, with an extremely limited historical range within Northwest Colombia [2] , [3] . Although no reliable estimates of historical population size exist, there must have been several tens of thousands in the 1960s, because 20–30,000 were captured and exported to the United States for use in biomedical experiments between the late 1960s and 1973 [3] , when the species was declared endangered. Although legal capture has been banned, illegal trafficking for use in the pet trade continues [2] . In addition to trapping, habitat destruction represents a major threat, as human populations expand and encroach in regions that were at one time sparsely inhabited [4] . Only one study [5] has quantified the scale of cotton-top tamarin habitat destruction, using visual interpretation of Landsat Thematic Mapper satellite images. They found a 31% decrease in the amount of available forest habitat between 1990 and 2000. Habitat destruction was noted even in protected areas: in the three national parks and protected areas where cotton-top tamarins have been observed, 42–71% of the forest was found to have been destroyed since they were designated [5] . Given the dramatic loss of habitat and the continued illegal capture of cotton-top tamarins, it is critical that we understand how these factors are impacting the remaining wild population. Our goal was to develop a census technique that would provide the first and only estimate of the current cotton-top tamarin population. However, censusing wild primate populations and estimating population numbers can be a difficult task because of challenges in species behaviour, field conditions and resource limitations. Four standard methods are territory mapping [6] , mark-recapture [7] , line transects for animals [8] and line transects for nests [9] , [10] , [11] , [12] , [13] . Territory mapping requires an enormous investment of resources to follow social groups long enough to estimate territory size accurately, and collect an adequate sample of groups over the species range. It also ignores non-territorial individuals. Mark-recapture is difficult for callitrichids, because they do not naturally have individually identifiable markings [14] , they are not distinguishable genetically [14] and once captured and marked (for example, with hair dye) they are difficult to recapture or resight because of a strong avoidance response. Traditional line transect methods do not work well for many small arboreal primates that tend to flee silently through the forest canopy before being counted [8] . Nest surveys work well for some ape species as they build large nests that are easily detected [9] , [10] , [11] , [12] , but callitrichids are not nest builders. For these reasons, although some studies have examined callitrichid species population densities at specific study sites [15] , [16] , [17] , there is only one reliable estimate of population size for any wild callitrichid population [18] . Cotton-top tamarins are highly territorial and frequently exchange territorial long call vocalizations with neighbouring groups [19] , [20] . They respond to playbacks of these vocalizations by approaching the stimulus source and vocalizing [21] , [22] . Counting the number of playback responses at a random sample of sites has been used as an index of population size in several mammals species [23] , [24] , but unless the distances from which responses come is known, this does not yield absolute population size. Such distances can be obtained for some species using a separate trial survey, in which playback experiments are performed on a sample of groups at known distances—a 'lure point transect' [25] —but initial trials on cotton-top tamarin groups indicated that tracking group locations to perform the experiment meant that they did not respond to the playback. Thus, we developed a 'lure strip transect' method that combines the idea of an acoustic lure with that of a strip transect—a sampling method that involves placing long, thin strips at random within the study area and counting all animals within the strips [26] . In our case, the strips were 200 m wide, and were surveyed by two field teams walking in parallel along the long edge of the strip, undertaking near-continuous playbacks to ensure that all animals within the transect were detected and counted. Strips were laid out using a systematic random grid in forest patches that had previously been identified as suitable habitat using analysis of satellite imagery [5] followed by field visits, and were also considered safe to work in (political instability meant that some areas were inaccessible). The number of animals counted within the surveyed strips was used to estimate population size by forest patch, administrative department and globally. Results from this study provided the first estimate of the wild population ( ∼ 7,394 individuals) and have been used in the development of long-term conservation strategies to protect this critically endangered primate and its forest habitat in Colombia. Test of assumptions The lure strip transect method relies on two main assumptions: that all animals within the strip are counted, and that none from outside are included. Previous studies [21] , [22] have shown that cotton-top tamarin groups respond to playbacks of territorial vocalizations by approaching the source and vocalizing. In developing the survey protocol, we undertook pilot trials in January 2005 at our long-term study site at Hacienda El Ceibal (Santa Catalina, Colombia). Using two habituated groups, in which location could be ascertained in advance using very high frequency telemetry without causing disturbance, trial playbacks indicated that the groups responded at a distance of 150–200 m, moving directly towards the sound source until all individuals in the group were easily within the range where they could be enumerated. Trials could only be performed twice on each group, as they quickly became used to the artificial sound source and stopped responding. For further validation, three unhabituated groups, in which group size and approximate location was known, trial transect surveys again resulted in all individuals in the group approaching close enough to be counted. Survey area Analysis of satellite imagery identified 14,534 km 2 of forested areas, spread over five administrative departments of Colombia ( Fig. 1 ). Of this, 4,019 km 2 was safely accessible to the field teams. Initial field visits in 2005 and 2006 showed that only 98.93 km 2 of this still contained forested habitat capable of supporting cotton-top tamarin populations, the majority of the rest having been cleared of forest, as the remotely sensed images were captured in 2000 (some were found to have been initially mis-classified). The remaining forest was made up of 43 patches, ranging in area from 0.18 to 17.35 km 2 . The systematic random grid design produced 301 transects to be surveyed in the forest patches and a 330 m buffer around them ( Fig. 2 ). Of these, 244 were surveyed, the others being missed because of either refusal by the landowner to grant access ( N = 8) or because they were in inaccessible terrain (for example, flooded at the time of the survey, recently clear cut or burned; N = 49). 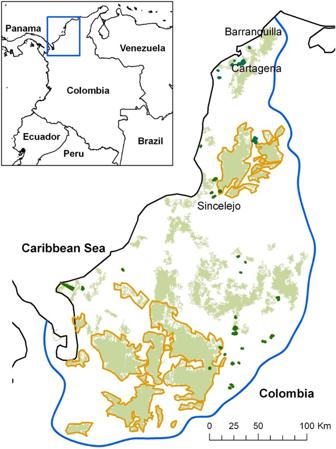Figure 1: Historic and current distribution of cotton-top tamarins in Colombia. Approximate historical range of cotton-top tamarin (blue line) within Colombia is far more extensive than areas identified as forest from Landsat satellite images in 2000 (shaded green). Of this, areas bordered by orange were not accessible to survey teams because of political instability. For the remaining areas, only the few fragments shown in dark green were found to be habitable forest when field teams visited during 2006–2007. The lure strip transect survey took place within these remaining fragments. Figure 1: Historic and current distribution of cotton-top tamarins in Colombia. Approximate historical range of cotton-top tamarin (blue line) within Colombia is far more extensive than areas identified as forest from Landsat satellite images in 2000 (shaded green). Of this, areas bordered by orange were not accessible to survey teams because of political instability. For the remaining areas, only the few fragments shown in dark green were found to be habitable forest when field teams visited during 2006–2007. The lure strip transect survey took place within these remaining fragments. 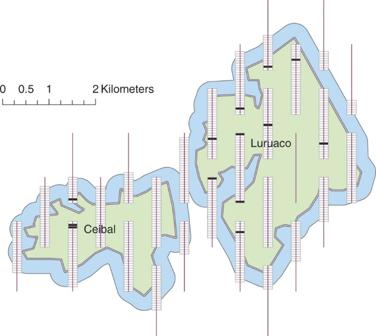Figure 2: Example of survey design. Two adjacent forest patches (green), with 30 m buffer (purple) and 330 m buffer (blue). The centre of each is indicated by a purple line. Rectangular boxes indicate surveyed line segments that were included in the analysis; all other segments were surveyed, but were discarded from the analysis because they were outside the buffered region, except for transect with no boxes which was inaccessible. Black boxes indicate segments in which cotton-top tamarins were encountered. Full size image Figure 2: Example of survey design. Two adjacent forest patches (green), with 30 m buffer (purple) and 330 m buffer (blue). The centre of each is indicated by a purple line. Rectangular boxes indicate surveyed line segments that were included in the analysis; all other segments were surveyed, but were discarded from the analysis because they were outside the buffered region, except for transect with no boxes which was inaccessible. Black boxes indicate segments in which cotton-top tamarins were encountered. Full size image Population estimates We encountered 178 groups of cotton-top tamarins (683 adults, 64 juveniles and 26 infants), of which 93 were within the transect strip. The resulting estimates of population size for each patch are given in Table 1 ; these were combined across patches to produce estimates by department and for all patches, given in Table 2 . The total population size estimate for all surveyed forest patches was 2,045 animals, with coefficient of variation of 13 and 95% confidence interval 1,587–2,633. Table 1 Estimates of population size ( N ) and other results by forest patch. Full size table Table 2 Estimates of population size ( N ) and other results for surveyed patches combined by department and across departments. Full size table Lastly, we obtained an approximate estimate of the global wild population size by scaling up the estimate of population size in the surveyed patches to account for the proportion of forested area identified by remote sensing that we could not safely survey, assuming population density in the surveyed and unsurveyed areas were equal. We were able to survey in 4,019 km 2 of the 14,534 km 2 forest area identified by remote sensing; hence, this amounted to multiplying our estimate for the surveyed patches by (14534/4019)=3.62. Because of uncertainties involved in this extrapolation, we did not attempt to derive variances on global population size. This gave an estimate of 7,394 animals. From our field trials, we believe that all individuals in a 200 m transect strip will be counted, or that failure to respond will be rare, so that any negative bias in the population estimate will be small. In the trials, groups moved straight towards the sound source, enabling those inside the strip to be distinguished from those outside. If there is substantial error in this assessment then this will cause a positive bias in the population estimate, because there is a larger area outside the strips than inside and, hence, more animals from outside will be counted in than animals from inside being counted out. However, we believe that, in practice, such errors in assessment are rare and any bias is again small. Additional assumptions were used in analysis, as detailed in the Methods section. As stated, we expect these assumptions to produce no bias in the population size estimates. However, because the variance estimator assumes completely random line placement, rather than systematic random, we anticipate that the estimates of variance are biased high—that is, that the population size estimates are more precise than that suggested by our coefficients of variation and confidence limits. Development of robust variance estimators for systematic survey designs would be helpful. The lure strip transect method is potentially useful for surveying other species for whom standard methods do not work or are not efficient, but who respond to playbacks. For some such species, trial playbacks on individuals or groups at known distances can be used to estimate a detection function and, hence, the lure point transect method [25] can be used. However, there are a significant number of species, including many small-bodied primates, for whom setting up trials involves undue disturbance or habituation. In these cases, if response is certain within some known range, lure strip transects can potentially produce robust results and are currently the only reliable method available. Our survey encompassed the historical range of the cotton-top tamarin, and therefore did not include any populations that have been introduced to the wild outside this range. For example, it is known that cotton-top tamarins were introduced into Panama near the border to Colombia, and it is thought that they have hybridized there with rufous-naped tamarin ( S. geoffroyi ) (A. Savage, personal observation). Other populations of released pets may exist on islands near Colombia, but these are likely very small and inbred. This study has provided important information to aid in the long-term conservation of the cotton-top tamarin. Since the wild population in the 1960s must have been at least several tens of thousands, our population estimate represents a substantial decline, and one that is likely to continue in the face of continuing habitat destruction and illegal capture. On the basis of these findings, cotton-top tamarins have been reclassified as critically endangered [1] and placed on the list of The World's 25 Most Endangered Primates 2008–2010 [27] . Efforts to establish protected reserves in northern Colombia are a priority. Larger remnant forest patches were identified during this research, as well as adjacent areas suitable for reforestation. A multi-stakeholder conservation plan has been developed, involving environmental authorities, non-governmental organizations, private land owners and local communities in creating and supporting the first protected area for cotton-top tamarins in northern Colombia. However, protecting habitat will not ensure the survival of the species if efforts are not made to stem the number of animals captured for the illegal pet trade or address the issues of removal of forest products for sale or consumption. Having population estimates by department allows us to examine how effective local conservation efforts are at protecting this critically endangered species for the future. Survey design To delineate the study area, remote-sensed spectral data collected in 2000 (Landsat 4, 5 and 7 Thematic Mapper satellite imagery) of the historic distribution of the cotton-top tamarin was used to identify forested areas [5] . Owing to political instability, some regions were not accessible to the field teams. For the rest, field teams visited every identified forest area between October 2005–January 2006 and January–February 2007. Many had been cleared of forest and no longer capable of supporting cotton-top tamarin populations; those remaining were mapped using a handheld global positioning system. A systematic grid of strip transects, with a random start point, was laid out over the study area. Each transect was 1.5 km long and 200 m wide, with the long axis oriented north–south. Transects were spaced 400 m apart in an 'offset' pattern ( Fig. 2 ). All transects that at no point came within 330 m of a forest patch were dropped. The reasons for the 330 m buffer were (1) mapping errors of up to 30 m could be expected and (2) cotton-top tamarins are occasionally seen foraging (for example, in trees along 'living hedges') up to 300 m outside the forest patch in which they are resident. Field methods Transects were surveyed only once, and surveys took place between 07:00 and 11:00 hours. At each transect, two field teams of four people traversed the long edges, using radio communication and global positioning system to ensure they remained parallel to one another and 200 m apart. The first individual in each team cut the trail, the second navigated and recorded data, the third carried a Bose Acoustic Wave Music System II that played adult cotton-top tamarin long calls (normal long calls and combination long calls [20] ; continuous play of 60 s of calls followed by 30 s silence, at 80 dB) recorded from captive animals at Disney's Animal Kingdom and the fourth watched and listened for cotton-top tamarins, and on making contact with animals, recorded location along the transect, number of animals (adult, juvenile and infant) and direction from which the group approached. This enabled those groups arriving from outside of the transect strip to be excluded from analysis. Data analysis overview Animal population size, N , was estimated using the formula where n s is the number of groups encountered, ŝ is the estimated population mean group size, a is the area covered by the transects and A is the area of the study region. Population size estimates were made for each forest patch, and these were then combined to produce estimates by administrative department and globally. Equation (1) contains two random components: group encounter rate ( n s /a ) and mean group size (ŝ); these were treated separately in the analysis as detailed below. An alternative approach would have been to analyze individual rather than group encounters: where n is the number of individuals encountered. However, the approach we took was expected to result in more precise estimates at the level of forest patch, because the encounter rate of groups ( n s /a ) showed less variation between transects within patches than encounter rate of animals ( n/a ), and mean group size ( s ) could be estimated more precisely by including groups that were detected during the survey, but were outside the transect strips, and potentially by pooling across forest patches. Estimation of encounter rate and variance by forest patch Animal density was much greater within forest patches than in the buffer area surveyed around the patches; hence, to reduce variance, we analyzed encounter rate data for each patch in two strata: core (the mapped patch, plus a 30 m buffer) and buffer (the area >30 m outside the mapped patches, but <330 m outside). There was one exception: in the Marimonda patch, open forest extended for up to 1 km around the core forest, and several groups were sighted within it; hence, a 1,030 m outer buffer limit was used there. During data collection, observers recorded where each sighting occurred along each transect line, dividing the 1.5 km lines into thirty 50 m segments. In calculating encounter rate for each line within each stratum, we assigned segments to either core or buffer strata, depending on where the majority of the segment area fell ( Fig. 2 ). Segments in which the majority of the area fell outside the core and buffer were discarded. Encounter rate for each stratum was then where n s,i is the number of groups recorded on the segments in line i and a i is the area of segments in line i . An initial estimate of variance in encounter rate for each stratum was calculated using the estimator R3 of Fewster et al . [28] This makes the mild assumption that variance in n s is proportional to the mean (that is, a Poisson-like model for counts, with overdispersion). We chose this estimator because it allows us to (1) produce more reliable estimates of variance for small forest patches by modelling the relationship between variance and mean and (2) estimate variance for patches not visited. Fewster et al . [28] showed that it is possible to construct variance estimators for systematic survey designs that produce lower (and more reliable) variance estimates, but it was not clear how to robustly do so here; hence, our variance estimates should be regarded as conservative (that is, biased high). Because some forest patches were very small, few lines were available in some strata to calculate variance, and hence these variance estimates were likely to be unreliable. To combat this, we modelled the relationship between vâr( n s ) (that is, a 2 vâr( n s / a ) and n s , extending the approach of Buckland et al . [29] (section 8.4.1)). 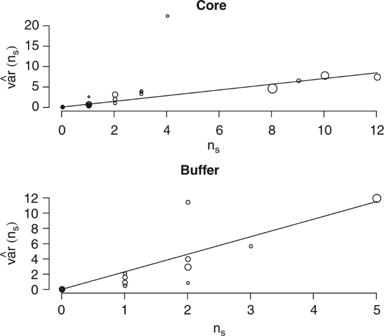Figure 3: Relationship between number of groups and variance in number of groups. The horizontal axis,ns, is the number of groups encountered for each forest patch and the vertical axis, vâr(ns), is the estimated between-transect variance in number of groups. Each circle represents one forest patch; the size of the circle indicates the area surveyed (that is, the regression weight). Core and buffer areas are shown separately, and the line shows the estimate from the best-fitting model (vâr(ns)∝ns—seeTable 4). We used weighted linear regression, with a forming the weight, and fit six models ( Table 3 ), selecting the one with the lowest Akiake Information Criterion. There was strong support for a model with vâr( n s ) proportional to n s , with a different slope parameter in the core and buffer areas ( Fig. 3 ). Slope estimates from this model were 0.70 (s.e. 0.06) in the core and 2.30 (s.e. 0.16) in the buffer. Values <1 indicate underdispersion relative to a homogeneous Poisson distribution and those >1 overdispersion; the value for the core could perhaps be explained by territorial spacing of cotton-top tamarin groups, whereas the overdispersion in the buffer by the very patchy nature of suitable habitat for movement outside of forested areas. Table 3 Model selection (Akaike Information Criterion) values for linear least-square models fit to encounter rate variance estimates. Full size table Figure 3: Relationship between number of groups and variance in number of groups. The horizontal axis, n s , is the number of groups encountered for each forest patch and the vertical axis, vâr( n s ), is the estimated between-transect variance in number of groups. Each circle represents one forest patch; the size of the circle indicates the area surveyed (that is, the regression weight). Core and buffer areas are shown separately, and the line shows the estimate from the best-fitting model (vâr( n s ) ∝ n s —see Table 4 ). Full size image Given the slope estimates, we predicted vâr( n s ) and hence vâr( n s / a ) for each forest patch. Before using these values in calculating variances on population size estimates by patch (see below), we applied the finite population correction factor [30] . This reduces the variance to account for the fact that for the part of each stratum covered by transects, population size is known (as it was counted), not estimated. The final estimate of variance for each stratum within forest patch, therefore, was where vâr( n s / a ) pred is the predicted variance from the regression model, a is the area surveyed in that stratum and A is the stratum area. In some patches, it was not possible to survey all of the planned transects. We assumed that these were missing at random with respect to animal density, and hence no special treatment was necessary during analysis. An exception was two patches that could not be surveyed at all (Buenos Aires (Sucre) and El Salado), and one where the core transects could not be surveyed (Aguas Prietas). We assumed that encounter rate on each stratum within these patches would have been equal to the average for the administrative department that they were in, and used equation (5) to predict the encounter rate variance without applying the finite population correction (that is, setting a =0). Estimation of mean group size To determine the appropriate level to estimate mean group size (by stratum (core/buffer) within forest patch, by patch or by administrative department), we performed a model selection exercise, using a zero-truncated Poisson regression. Input data were group sizes of all groups detected while moving along transect lines, both inside and outside the transect strip. Potential factor covariates were patch stratum (core/buffer), patch and department. The selected model was that with the lowest Akiake Information Criterion: this was the model with mean group size pooled across all data ( Table 4 ). Table 4 Model selection (Akaike Information Criterion) values for zero-truncated Poisson regression models fit to group size data. Full size table Estimation of population size and variance Population size for each stratum within patch was estimated using equation (1), using estimates of encounter rate and mean group size derived as described in previous sections. Variance was estimated using the delta method [31] 95% confidence intervals were obtained by assuming that N is a log-normal random variable (for example, Buckland et al . [29] , section 3.6.1). Population size by patch was estimated as the sum of the estimates from the core and buffer strata. Variance was again estimated using the delta method, with cluster size variance estimated as given above and encounter rate variance estimated as the sum of the stratum-level encounter rate variances. This ignored the non-independence in encounter rates, generated when the same transect occurs in both core and buffer strata, and will result in slight overestimation of variance; however, given the large number of transects overall, and the large difference in density between core and buffer, this effect should be negligible. How to cite this article: Savage, A. et al . Novel survey method finds dramatic decline of wild cotton-top tamarin population. Nat. Commun. 1:30 doi: 10.1038/ncomms1030 (2010).